Weyl fermions and spin dynamics of metallic ferromagnet SrRuO3 Weyl fermions that emerge at band crossings in momentum space caused by the spin–orbit interaction act as magnetic monopoles of the Berry curvature and contribute to a variety of novel transport phenomena such as anomalous Hall effect and magnetoresistance. However, their roles in other physical properties remain mostly unexplored. Here, we provide evidence by neutron Brillouin scattering that the spin dynamics of the metallic ferromagnet SrRuO 3 in the very low energy range of milli-electron volts is closely relevant to Weyl fermions near Fermi energy. Although the observed spin wave dispersion is well described by the quadratic momentum dependence, the temperature dependence of the spin wave gap shows a nonmonotonous behaviour, which can be related to that of the anomalous Hall conductivity. This shows that the spin dynamics directly reflects the crucial role of Weyl fermions in the metallic ferromagnet. The spin dynamics in magnets is an important subject studied for many decades. Early studies are based on the spin Hamiltonians where the electronic states are indirectly reflected in the magnetic parameters [1] . Recently, microscopic understanding starting from the electronic band structures has become a realistic target with the help of advanced first-principles calculations [2] , [3] , [4] . In ferromagnets, repulsive Coulomb interaction between electrons results in an exchange splitting J ex between bands with up () and down () spins, which produces spontaneous magnetization, as shown in Fig. 1a . Therefore, the band crossings ɛ n ( k )= ɛ m ( k ) ( n m ) between the different bands ( n th and m th bands), where ɛ n ( k ) and ɛ m ( k ) are the momentum ( k ) dependence of the energy bands of the corresponding states, occur on two-dimensional surface in the three-dimensional momentum space. In the presence of spin–orbit interactions, λ 1 ( k ) and λ 2 ( k ), that mix different spin components and give the off-diagonal matrix elements, the band crossings turn into anti-crossings with the gap as indicated by the red curve in Fig. 1a . 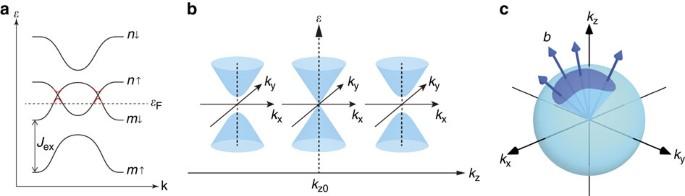Figure 1: Schematic band structure and Weyl fermion in ferromagnets. (a) The energy (ɛ) dispersions of up () and down () spin bands with the exchange splittingJex.ɛFis the Fermi energy. The band crossingsɛn(k)=ɛm(k) occur when the overlap of the up and down spin bands are finite. In the presence of the spin–orbit interaction, which mixes the up and down spins, the band crossings turn into the anti-crossings with the gap opening (red curve). (b) Band structure near the Weyl pointk0. The band dispersions with fixedkzare shown in thekx–kyplane. The gap closes at the Weyl pointk=k0. (c) Distribution of the emergent magnetic fieldb(k) near a Weyl point. The flux penetrating the areaSis given by the solid angle subtended byS, and the total flux is 2πη. Therefore, Weyl fermion acts as a monopole or anti-monopole of the emergent magnetic field depending on the chiralityη=±1. More explicitly, the effective Hamiltonian reads Figure 1: Schematic band structure and Weyl fermion in ferromagnets. ( a ) The energy ( ɛ ) dispersions of up () and down () spin bands with the exchange splitting J ex . ɛ F is the Fermi energy. The band crossings ɛ n ( k )= ɛ m ( k ) occur when the overlap of the up and down spin bands are finite. In the presence of the spin–orbit interaction, which mixes the up and down spins, the band crossings turn into the anti-crossings with the gap opening (red curve). ( b ) Band structure near the Weyl point k 0 . The band dispersions with fixed k z are shown in the k x – k y plane. The gap closes at the Weyl point k = k 0 . ( c ) Distribution of the emergent magnetic field b ( k ) near a Weyl point. The flux penetrating the area S is given by the solid angle subtended by S , and the total flux is 2 πη . Therefore, Weyl fermion acts as a monopole or anti-monopole of the emergent magnetic field depending on the chirality η =±1. Full size image with 2 × 2 Pauli matrices σ =( σ 1 , σ 2 , σ 3 ), and the gap is given by . This gap closes when the three coefficients of the Pauli matrices σ ’s are zero in equation (1), which can be satisfied by tuning the three components of the momentum k at some k 0 in three dimensions. Figure 1b shows this situation, where the energy dispersions at each fixed k z and the gap closes at k = k 0 . Expanding equation (1) with respect to k – k 0 , one obtains H = ηv ( k – k 0 )· σ with the momentum k being appropriately redefined. Here v is the velocity and η =±1 determines the chirality. This is nothing but the Weyl fermion and k 0 is called Weyl point, which is ubiquitous in magnets as long as the band overlaps of both spin components are finite. It has been pointed out that the band crossing of the form in equation (1) is of crucial importance for the Berry curvature; it acts as a source or sink (monopole) of the emergent magnetic field b ( k ). More explicitly, as shown in Fig. 1c , and the flux integral over the surface enclosing k 0 is 2 πη . This emergent magnetic field gives the anomalous velocity and Hall current in the presence of the external electric field, which is the origin of the intrinsic anomalous Hall effect in ferromagnets: that is, σ xy can be written as the integral of the Berry phase curvature (the gauge field) over the occupied electronic states [5] , [6] , [7] , [8] . The anomalous Hall effect emerging in the ferromagnetic phase of SrRuO 3 has been analysed from this viewpoint, where σ xy shows nonmonotonous dependence on the magnetization. We note that this anomalous Hall effect can be well reproduced by a first-principles calculation. In the ferromagnetic phase of SrRuO 3 , also a tight-binding model reveals that a number of Weyl points are produced in the first Brillouin zone by the above-mentioned process [9] . Therefore, the origin of the Berry curvature resulting in the nonmonotonous σ xy in SrRuO 3 is Weyl fermions as magnetic monopoles [6] , [7] , [8] , [9] , [10] . The optical Hall conductivity σ xy ( ω ) in the terahertz region also supports the presence of Weyl fermion within the range of 5 meV near the Fermi energy [11] . Recently, several materials have been theoretically proposed and experimentally studied, where Weyl fermions are located exactly at the Fermi energy and govern the transport phenomena, that is, Weyl semimetals [12] , [13] , [14] , [15] , [16] , [17] , [18] . For example, the large magnetoresistance is discussed from the viewpoint of chiral anomaly. We note that the previous studies are, however, restricted mostly to the transport properties, and the influence of Weyl fermions on other phenomena are unexplored. In this paper, we report the fingerprint of Weyl fermions and magnetic monopoles in the spin dynamics of SrRuO 3 . It has been recognized that SrRuO 3 is a rare example of 4d band ferromagnetic metal with a pseudo-cubic perovskite crystal structure, and the ferromagnetism has been extensively studied [19] , [20] , [21] . Recently, a large spin wave gap was observed in SrRuO 3 (ref. 22 ), whereas La 0.8 Sr 0.2 MnO 3 , a ferromagnet having a similar pseudo-cubic structure, showed no spin wave gap [22] . Although the large magnetic anisotropy in SrRuO 3 is one of remarkable features, no anomaly in the temperature dependence of the magnetic anisotropy has been found in the static properties [19] , [20] , [21] , [23] . We show that Weyl fermions play a crucial role in the spin dynamics by measuring the temperature dependence of spin waves in SrRuO 3 . Spin waves observed by neutron Brillouin scattering (NBS) We have measured small momentum magnetic excitations in a polycrystalline sample of SrRuO 3 by NBS experiments, namely inelastic neutron scattering (INS) experiments near the forward direction. In case that a sizable single crystal is not available, NBS is the most appropriate magnetic INS method for studying the spin dynamics. The state-of-the-art instrument (High-Resolution Chopper Spectrometer, HRC) at intense pulsed neutron scattering facilities like J-PARC (Japan Proton Accelerator Research Complex) has provided an opportunity for the present study approaching the kinematical constraint of the neutron scattering by providing high-energy neutrons of sub eV region. Typical data of the observed INS spectra are shown in Fig. 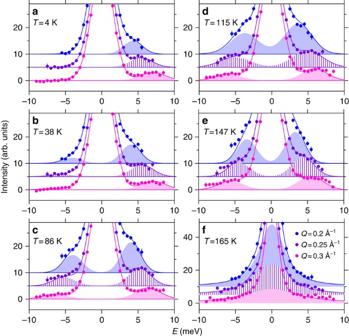Figure 2: Background subtracted INS spectra in SrRuO3. Observed spectra are displayed as a function ofEat severalQvalues (0.2, 0.25, 0.3 Å−1) for selectedT(a: 4 K,b: 38 K,c: 86 K,d: 115 K,e: 147 K,f: 165 K). Spectra are shifted by a constant to aid the eye. The vertical bars represent statistical errors determined from the square root of neutron counts. The solid lines are fitted curves to the observed spectra, and the shaded areas are magnetic components. 2 , and were analysed by using the scattering functions I ( Q , E ) expressed as follows: Figure 2: Background subtracted INS spectra in SrRuO 3 . Observed spectra are displayed as a function of E at several Q values (0.2, 0.25, 0.3 Å −1 ) for selected T ( a : 4 K, b : 38 K, c : 86 K, d : 115 K, e : 147 K, f : 165 K). Spectra are shifted by a constant to aid the eye. The vertical bars represent statistical errors determined from the square root of neutron counts. The solid lines are fitted curves to the observed spectra, and the shaded areas are magnetic components. Full size image where E and Q is the energy and momentum transfers of neutrons, respectively. Equation (2) presents the spectrum for the spin waves with energy E S at temperature T below the ferromagnetic transition temperature T C (=165 K), and equation (3) corresponds to the paramagnetic scattering with the energy width Γ at T = T C . The magnetic form factor of spin component can be approximated to be F ( Q )=1 in the present small Q range. A S ( Q ) and A C ( Q ) represent the other Q dependence in the scattering intensity. The thermal population factor is given by n +1=[1–exp(− E / k B T )] −1 with the Boltzmann constant k B . Each scattering function is the form convoluted with the instrumental resolution, and contains the elastic scattering component B ( Q , E ). Δ E is the energy resolution and W is the energy width of spin waves determined from the instrumental resolution. Δ E and B ( Q , E ) are determined experimentally. The quantities, A S , A C , E S and Γ, are determined by the standard least square fitting procedure, as shown in Figs 2 and 3 . 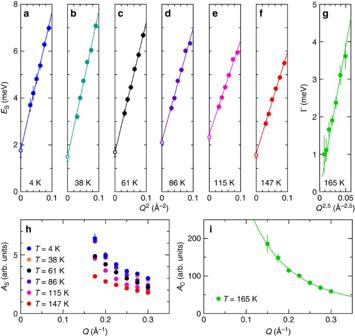Figure 3: Parameters in scattering function for spin waves and critical scattering in SrRuO3. (a–f) Spin wave energyESand (h) intensityAS(Q) are plotted inQfor selectedTbelowTC=165 K. The lines in (a–f) are fitted to the quadratic dispersion relation, and the open circles atQ=0 Å−1are the spin wave gapEgobtained by the fit. (g) Energy width Γ and (i) intensityAC(Q) of the paramagnetic scattering atT=TCare plotted inQ. The lines ingandiare the fitted curves to the dynamical scaling law. The vertical bars represent statistical errors, some of them are smaller than the sizes of the marks. Figure 3: Parameters in scattering function for spin waves and critical scattering in SrRuO 3 . ( a – f ) Spin wave energy E S and ( h ) intensity A S ( Q ) are plotted in Q for selected T below T C =165 K. The lines in ( a – f ) are fitted to the quadratic dispersion relation, and the open circles at Q =0 Å −1 are the spin wave gap E g obtained by the fit. ( g ) Energy width Γ and ( i ) intensity A C ( Q ) of the paramagnetic scattering at T = T C are plotted in Q . The lines in g and i are the fitted curves to the dynamical scaling law. The vertical bars represent statistical errors, some of them are smaller than the sizes of the marks. Full size image The spin wave energies E S can be well fitted to the simple dispersion relation for ferromagnetic spin waves E S ( Q )= E g + DQ 2 , which is clearly extrapolated to the finite spin wave gap E g ∼ 2 meV, as shown in Fig. 3a–f . The peak intensities A S ( Q ) in Fig. 3h increase as Q gets reduced, which suggests that the magnetic excitations contain another component, that is, orbital moment, other than spin. The large E g emerges due to the spin–orbit interaction as described below. We note that the increase in A S ( Q ) at low Q can be in accord with the spreading of the orbital component in real space. As shown in Fig. 4a , D decreases as T increases, that is a normal behaviour observed in both localized electron systems and itinerant electron systems [24] . On the other hand, E g shows nonmonotonous thermal evolution. The finite value of E g indicates an internal magnetic field acting on the system. 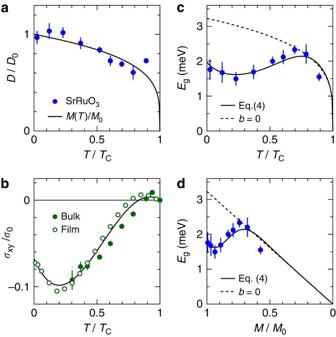Figure 4: Stiffness constant and spin wave gap in SrRuO3. (a) Stiffness constantD, (b) anomalous Hall conductivityσxy/σ0with σ0=9.9 × 102Ω−1cm−1, (c) spin wave gapEgas a function ofT/TCand (d)Egas a function ofM(T)/M0. The vertical bars inaandcrepresent the statistical errors of the measured values. The solid line inais the measured curve ofM(T)/M0. The experimental data ofσxy(T) for the bulk sample and those for the film sample scaled to the bulk samples are plotted with an empirical curve (solid line) to expressσxy(T) for both samples inb, where the vertical bars represent experimental errors. The solid lines incanddare the fit to equation (4) witha=3.2 meV andb=−9.5, and the dashed lines incanddare the calculated curves witha=3.2 meV andb=0, by using the empirical curve forσxy. It should be noted thatD(T) andEg(T) are proportional to magnetizationM(T) in the strong correlation limit. Figure 4: Stiffness constant and spin wave gap in SrRuO 3 . ( a ) Stiffness constant D , ( b ) anomalous Hall conductivity σ xy / σ 0 with σ 0 =9.9 × 10 2 Ω −1 cm −1 , ( c ) spin wave gap E g as a function of T / T C and ( d ) E g as a function of M ( T )/ M 0 . The vertical bars in a and c represent the statistical errors of the measured values. The solid line in a is the measured curve of M ( T )/ M 0 . The experimental data of σ xy ( T ) for the bulk sample and those for the film sample scaled to the bulk samples are plotted with an empirical curve (solid line) to express σ xy ( T ) for both samples in b , where the vertical bars represent experimental errors. The solid lines in c and d are the fit to equation (4) with a =3.2 meV and b =−9.5, and the dashed lines in c and d are the calculated curves with a =3.2 meV and b =0, by using the empirical curve for σ xy . It should be noted that D ( T ) and E g ( T ) are proportional to magnetization M ( T ) in the strong correlation limit. Full size image The T dependence of E g is nonmonotonous and clearly differs from that of the spontaneous magnetization M . A magneto-optical measurements showed the ferromagnetic resonance (FMR) frequency at 250 GHz almost independent of T at T <80 K (ref. 23 ); this also differs from M ( T ). Both E g and the FMR frequency show the anomalous T dependence. The observed E g =1.5–2.1 meV at low T including the error bars is of the comparable magnitude as E g ∼ 1 meV estimated by the FMR frequency of 250 GHz. The anisotropy energy of K ∼ 12 T estimated by the bulk magnetization [21] is comparable to these values. At zero temperature, is given both in the strong and weak correlation cases; if we use the value for a powder sample [25] , we obtain E g ∼ 1 meV. The dipole interaction can also contribute to the spin wave gap at the zone centre, which is directly observed by the FMR and Brillouin light scattering. Such gap is 0.03 meV for yttrium iron garnet film [26] , and we anticipate it to be smaller for SrRuO 3 having smaller magnetic moment than the yttrium iron garnet film. It should be noted that, in the NBS using a polycrystalline sample, E g is extrapolated from the dispersion observed at finite Q by mapping onto the simple spin Hamiltonian neglecting such a small dipole interaction. The nonmonotonous T dependence of the anomalous Hall conductivity σ xy of SrRuO 3 was discussed from the viewpoint of Weyl fermions, that is, magnetic monopoles in the momentum space [6] , [8] , [10] . Similarly, Weyl fermions are expected to produce the nonmonotonous T dependence of the spin dynamics as well. As discussed below, E g is expected to be fitted by the following formula; Here, σ 0 = e 2 / ha 0 =9.9 × 10 2 Ω −1 cm −1 ( a 0 being the lattice constant of SrRuO 3 ) is used as a normalization factor for σ xy . As shown in Fig. 4c,d , the nonmonotonous T dependence of E g can be well reproduced by using the parameter of a =3.2 meV and b =−9.5. For M ( T )/ M 0 and σ xy ( T )/ σ 0 , we used the experimental results (see the Methods for details). Now we sketch the theoretical background of equation (4) (see the Methods for details). The spin wave at the zero momentum is described by the action obtained by integrating over the electrons as (ref. 27 ) where the first term with the coefficient α is the integrand represent of the Berry phase, whereas the second term is the spin anisotropy energy. Then spin wave gap E g ( T ) is given by the ratio K / α . The main idea is that the Weyl fermions contribute resonantly to α as in the case of σ xy because of the small energy denominator, although the former takes the finite value α 0 even without the spin–orbit interaction, whereas the latter comes solely from the spin–orbit interaction (see the Methods for details). Assuming a single Weyl fermion near the Fermi energy, as suggested by the terahertz optical spectroscopy [11] , there is a one-to-one correspondence between the spin operators and current operators. Therefore, the contribution α 1 to the coefficient α from the Weyl fermion is given by λσ xy with λ being a constant. Since (see the Methods for details), we obtain , which is equivalent to equation (4). Here the temperature-independent anisotropy energy K is assumed, which is justified down to T ∼ 40 K by the magnetization curve measurement [28] . To conclude, the nonmonotonous temperature dependence of the spin wave gap is unveiled by NBS in SrRuO 3 , which is related to its nonmonotonous anomalous Hall effect through the Weyl fermions near the Fermi energy. This result has revealed the connection between the transport and dynamical magnetic properties through the enhanced spin-orbit coupling effect. NBS employed here has the large potentiality. It can provide the detailed information of the generalized magnetic susceptibility in the small Q -region in addition to the energy of the magnetic excitations, which we focused in the present paper. NBS will thus provide a powerful method to solve unsettled issues in dynamical magnetism, including a role of orbital component in the magnetic fluctuation. Materials The sizable single crystals of SrRuO 3 necessary for INS experiments have never been synthesized so that the spectroscopic studies must be performed using powder (polycrystalline) samples. We prepared polycrystals of SrRuO 3 (73 g) by the well-established method of synthesis [25] , and the high quality of the sample was confirmed by our subsequent bulk measurements. The crystal structure with a single phase was confirmed by the X-ray diffraction. The magnetization measurement under the low magnetic field ( H =10 Oe) is well fitted to m ( T )= m 0 (1–( T / T C ) a ) b , as shown in the inset of Fig. 5a , and the ferromagnetic transition temperature was determined to be T C =165 K. This value of T C is the highest in the powder forms and comparable to that of the single-crystal forms. 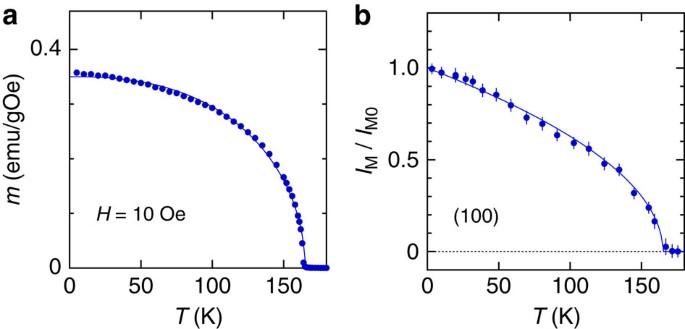Figure 5: Determination of ferromagnetic transition temperatureTCand critical exponentβ. (a) The ferromagnetic transition temperatureTC(=165 K) is estimated from the temperature dependence of the low-field magnetization. (b) The temperature dependence of magnetic Bragg scattering at (100) is well fitted toIM(T)=IM0(1–T/TC)2β, and the critical exponent is determined to beβ=0.25±0.01 by usingTC=165 K. Figure 5: Determination of ferromagnetic transition temperature T C and critical exponent β . ( a ) The ferromagnetic transition temperature T C (=165 K) is estimated from the temperature dependence of the low-field magnetization. ( b ) The temperature dependence of magnetic Bragg scattering at (100) is well fitted to I M ( T )= I M0 (1– T / T C ) 2 β , and the critical exponent is determined to be β =0.25±0.01 by using T C =165 K. Full size image The elastic neutron scattering from the magnetic Bragg reflection at (100) was observed on the HRC (see below) with E i =12.5 meV. The observed intensity is the sum of the T -dependent magnetic component I M and the constant nuclear component I N , and thus, well fitted to I ( T )= I M + I N = I M0 (1– T / T C ) 2 β + I N with the above-obtained value of T C =165 K by parameterizing β , I M0 and I N , as shown in Fig. 5b , where I M / I M0 =( I ( T )– I N )/ I M0 is plotted. The obtained critical exponent β =0.25±0.01 agrees well with that from the early neutron diffraction experiment [29] . Therefore, we used the T dependence of the saturation magnetization, M ( T )/ M 0 =(1– T / T C ) β with these values of T C and β for the analysis of D ( T ) and E g ( T ). The stiffness constant D ( T ) at T =4–130 K was fitted with D 0 (1– T / T C ) β and D 0 was obtained to be 62 meV. For the transport measurement, the powder sample of SrRuO 3 obtained in the same batch as that for the INS experiments was sintered by high-pressure spark plasma sintering and patterned in Hall bar geometry using conventional photo-lithography and Ar ion dry-etching. The Hall resistivity ρ H was measured together with the longitudinal and transverse resistivities, ρ xx and ρ yx , as a function of T under an applied magnetic field. The anomalous resistivity ρ yx was determined after subtracting the ordinary Hall contribution from the measured ρ H , and the transverse conductivity σ xy was determined as ρ yx /( ρ xx 2 + ρ yx 2 ) ≅ ρ yx / ρ xx 2 , and plotted in Fig. 4b as the bulk sample. The error bars of σ xy for the bulk sample are large at low temperatures because of very small values of resistance. On the other hand, the error bars of σ xy for the film sample are relatively small because of high resistance and well-defined shape of the Hall bar [10] . We also plotted σ xy for the film sample [10] , which was scaled to the bulk data by a factor of 0.61. The reduction factor of 0.61 was determined by minimizing the difference ( χ 2 ) between the bulk data and the film data. An empirical formula was established to express σ xy ( T ) for both the film and the bulk samples, as indicated with the solid line in Fig. 4b . For the analysis of E g ( T ), we used the empirical formula for σ xy ( T )/ σ 0 , where σ 0 = e 2 / ha 0 =9.9 × 10 2 Ω −1 cm −1 with a 0 =3.9 Å being the atomic distance, e being the elementary charge and h being the Planck’s constant. NBS and data analysis To observe ferromagnetic excitations in a polycrystalline sample, we have applied the NBS method by using the HRC installed at the Materials and Life Science Experimental Facility, J-PARC [30] . On the HRC, neutron beams extracted from the pulsed neutron source are monochromatized by a Fermi chopper (the incident neutron energy ( E i ) is selected) and are incident upon the sample. Scattered neurons, of which energy transfer ( E ) is determined from the time-of-flight, are collected with a detector system covering the scattering angles continuously. By utilizing high-energy (sub eV) neutrons with the short pulses realizing the high-energy resolution of Δ E / E i ∼ 2% on the HRC, one can perform NBS experiments, that is, INS experiments near to the forward direction like the conventional optical Brillouin scattering method [22] , [30] . Normally, a sizable single crystal is required for INS experiments. However, excitations near to the zone centre, where scattering intensities remain even by the powder average of the dynamical structure factor, can be detected by the NBS. To measure the spin wave dispersion relation for SrRuO 3 , we selected E i =100 meV. Then, the transferred energy E reaches to higher than 10 meV with the energy resolution Δ E =2 and 3.4 meV and the transferred momentum Q approaches down to ∼ 0.15 and 0.175 Å −1 , respectively, by using the detecting system that covers the scattering angles down to 0.6°. The condition with Δ E =3.4 meV provides the peak intensity of the excitation spectrum twice that with Δ E =2 meV. Several experimental improvements have made the NBS methods feasible in the practical level for our studies: they include the short-pulse and the high-energy neutrons with higher flux provided by the intense pulsed neutron source as well as the lower background at low angles. Using this new state-of-the-art instrument HRC, we could achieve the data quality equivalent to that by INS measurements with single crystals [22] . These improvements in the instrumentation made it possible for us to get access to the current ( Q , E ) space, which is essential for this study. The HRC provides the highest resolution of its class in the ( Q , E ) space for the present study. We measured the INS spectra at T =4, 20, 38, 61, 86, 115 and 147 K with the Δ E =3.4 meV condition, and at T =4, 100, 130 and 165 K with the Δ E =2.0 meV condition. It should be noted that the spin wave dispersion relation obtained at T =4 K with the Δ E =3.4 meV condition was identical to that with the Δ E =2.0 meV condition. The scanned data without the sample was defined as the background, which was subtracted from the raw data after normalizing by the exposure time of the data acquisition. The E dependence of the background-subtracted intensities were well fitted with equation (2) or (3). The functional form of the elastic scattering B ( Q , E ) in equations (2) and (3) is almost described by a Gaussian function centred at E =0 meV with Δ E being the full-width at half-maximum, however, it has a tiny tail at the negative E side. The neutrons are emitted from the neutron source with a time distribution, and the tail originates from the neutrons with higher energies than E i emitted later than the time origin of the time-of-flight and transmitted through the time window of the Fermi chopper. The value of Δ E and the shape of the tail in B ( Q , E ) were determined by measuring the shape of the incoherent elastic scattering at low T and higher Q , where the elastic peak is well separated from the spin wave peaks. As the elastic component consists of the incoherent elastic scattering and the Bragg scattering at the zone centre, B ( Q , E ) decreases as Q increases and becomes constant. The peak value of B ( Q , E ) can be determined as the peak intensity of the Gaussian component in each spectrum. It should be noted that Δ E is independent of Q . The spin wave components could be described by the Gaussian function with the width W in equation (2), which was estimated from Δ E and the influence of the Q resolution via the spin wave dispersion as follows [22] , [31] , where d E S /d Q =2 DQ , and Δ Q =0.12 Å −1 is estimated from the instrumental geometry [22] . The value of D in Fig. 4a was used after some iterations. The excitation energy width finer than W cannot be determined experimentally. As the tail in B ( Q , E ) is much smaller than the peak intensity of B ( Q , E ), the resolution-limited scattering can be approximated to a Gaussian scattering function with the width W determined by the instrumental resolution, neglecting the small contribution of the tail. Similar to this, the resolution function with which the Lorentzian component is convoluted for the spectrum at T = T C can be approximated to a Gaussian scattering function with Δ E , as shown in equation (3). The spin wave energies E S decrease upon heating and eventually go to zero at T C . The spectra also change their nature from the Gaussian function for spin waves to the Lorentzian function centred at E =0 meV for the paramagnetic spin fluctuations, as shown in Fig. 2 . The scattering function at T = T C is typical of the critical scattering observed in metallic ferromagnets [32] : the power law Γ= γQ 2.5 clearly holds with γ =76 meV Å 2.5 , and the Q dependence of intensity A C ( Q ) is well fitted to the functional form of the critical scattering ( Q −2 ) convoluted with the instrumental resolution, as shown in Fig. 3g,i . This indicates that the spectra observed at T < T C are of spin waves. In the case of ferromagnetic spin waves, the dispersion relation normally follows the Q 2 law ( E S ( Q )= DQ 2 + E g ) independently of the crystalline orientation in a small Q region for cubic or isotropic lattices. In fact, spin waves in the single crystalline sample of the nearly cubic perovskite La 0.8 Sr 0.2 MnO 3 show the isotropic Q 2 law ( E g =0 meV) at Q ≤0.3 Å −1 , although the dispersion curve along [001] bends down to lower energies than the [111] curve at Q >0.3 Å −1 (ref. 33 ). The dispersion relation at Q ≤0.3 Å −1 observed by the NBS on the HRC using a polycrystalline sample of La 0.8 Sr 0.2 MnO 3 was identical to that obtained by using the single crystalline sample [22] . Although the crystal structure of SrRuO 3 is orthorhombic, similar to La 0.8 Sr 0.2 MnO 3 , it can be approximated to be cubic with the lattice constant of 3.9 Å within the present instrumental resolution. We applied this established experimental technique to the present study of the spin dynamics in SrRuO 3 . 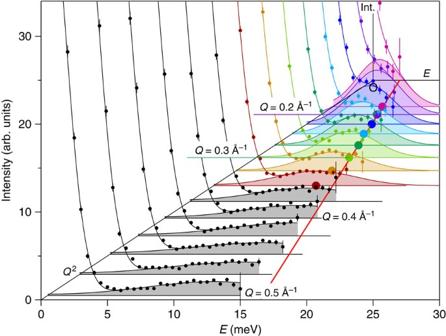Figure 6: Background subtracted INS spectra in SrRuO3observed atT=4 K on the HRC. INS spectra are plotted atQ=0.175–0.5 Å−1at a step of 0.025 Å−1, which are indicated with small solid circles with vertical bars presenting the statistical errors. Each spectrum was fitted with equation (2) by using the calculated resolution widthWforQ≤0.3 Å−1and by parameterizingWforQ>0.3 Å−1. The solid lines are the fitted curve to the spectrum, and the shaded areas are the spin wave components obtained by the fit. The determined spin wave peak positions are plotted with large circles. The different colours correspond to the differentQvalues. The red line indicates the spin wave dispersion with theQ2law determined forQ≤0.3 Å−1. Figure 6 shows the INS spectra in SrRuO 3 observed on the HRC at Q =0.175–0.5 Å −1 at a step of 0.025 Å −1 . The spin wave peak positions for SrRuO 3 were well defined and described by the Q 2 law at Q ≤0.3 Å −1 , however, deviated from the Q 2 law at Q >0.3 Å −1 . Furthermore, the spectra became much broader at Q ⩾ 0.375 Å −1 and the peak positions could not be accurately determined. Therefore, we confirmed that the spin wave dispersion can be approximated to the Q 2 law by using data for Q ≤0.3 Å −1 . All our analyses reported here are based on the data collected for Q ≤0.3 Å −1 . Figure 6: Background subtracted INS spectra in SrRuO 3 observed at T =4 K on the HRC. INS spectra are plotted at Q =0.175–0.5 Å −1 at a step of 0.025 Å −1 , which are indicated with small solid circles with vertical bars presenting the statistical errors. Each spectrum was fitted with equation (2) by using the calculated resolution width W for Q ≤0.3 Å −1 and by parameterizing W for Q >0.3 Å −1 . The solid lines are the fitted curve to the spectrum, and the shaded areas are the spin wave components obtained by the fit. The determined spin wave peak positions are plotted with large circles. The different colours correspond to the different Q values. The red line indicates the spin wave dispersion with the Q 2 law determined for Q ≤0.3 Å −1 . Full size image Theoretical analysis The basic facts about theories of spin wave dispersion and the effects of the Weyl fermions are summarized here. First, the T dependence of the stiffness constant D without the spin–orbit interaction has been studied theoretically both in the strong and weak correlation limits. In the strong correlation case, the spin wave is discussed in terms of the Heisenberg spin Hamiltonian . The linearized equation of motion with respect to S + = S x + iS y reads which results in , where Q =| q | for small q =( q x , q y , q z ) ( Q ≤0.3 Å −1 in the present case). On the other hand, in the weak correlation limit, although random phase approximation predicts the diverging D ( T ) towards T C (ref. 34 ), the self-consistent renormalization theory predicts the vanishing D ( T ) as T → T C (refs 35 , 36 ). Experimentally, D ( T ) for a metallic ferromagnet Ni 3 Al, for instance, decreases to zero as T increases to the transition temperature T C . This behaviour is consistent with both the self-consistent renormalization theory [35] , [36] , and also the Heisenberg model [24] . In the weak correlation limit, the spin wave dispersion is determined by the generalized spin susceptibility χ +− ( q , ω ) of electrons as given as follows [34] , with where is the generalized spin susceptibility without the electron–electron interaction, f ( ɛ ) is the Fermi distribution function and is the energy dispersion of up (down) spin with U being the electron–electron interaction. By solving the equation , one can obtain the spin wave dispersion ω ( q ). Although the detailed form depends on ɛ ( k ), one can consider the expansion of χ +− ( q , ω ) with respect to ω and q . The coefficient α 0 of ω is , whereas that of q 2 is near the transition temperature T C (ref. 34 ). Next, we consider the effects of the spin–orbit interaction. In the strong correlation limit, it introduces the spin anisotropy term , which adds the gap to the spin wave dispersion ω ( q ). Although experiments determining the spin wave gap have been often reported, the reports on its temperature dependence are very few. In the case of ferromagnets, the temperature dependence of the spin wave gap is hardly detected, because a ferromagnet having a crystal structure with high symmetry normally shows gapless spin wave. In the case of antiferromagnets, spin wave gap can be enhanced by the exchange interaction J as . The antiferromagnetic resonance frequency, that is a spin wave gap in antiferromagnet and is also proportional to , shows a monotonous temperature dependence as a function of the magnetization for insulating antiferromagnets such as MnF 2 (ref. 37 ) and MnO (ref. 38 ). The spin wave gap shows a monotonous temperature dependence as a function of the magnetization even for a metallic antiferromagnet γFeMn (ref. 39 ). Equation (9) should be generalized to include the spin–orbit interaction in the electronic band structure, where n,m are the band indices including the pseudospin. Equation (10) usually has a complex form, but one can consider the expansion with respect to ω and q as discussed above. The zero-th order term χ +− ( 0 ,0)– χ zz ( 0 ,0) determines the anisotropy K , which is basically independent of T near T C , that is, it can be defined even in the normal phase. On the other hand, when we expand with respect to ω as the linear order term in ω contains the square of the energy denominator, and is hence sensitive to the Weyl fermions [27] . Now we discuss how equation (4) is derived theoretically based on the Weyl fermion. The spin dynamics is described by the effective action A for the spin fluctuation field S α obtained by integrating over the electronic degrees of freedom as [27] Where is the correlation function of the conduction electron spin σ α . We are interested in the action A 0 for the uniform component ( q =0), which is given by equation (5), where the coefficient α of the Berry phase term is given by , and K represents the spin anisotropy energy. Most of the contribution to α comes from the bands not largely influenced by the spin–orbit interaction, that is, α 0 , and nontrivial contribution α 1 comes from Weyl fermions. As described above, . The contribution α 1 from the Weyl fermion is proportional to σ xy , as shown below. The Hamiltonian in equation (1) is rewritten as , where f a ( k ) is expanded near the band crossing point k 0 as . One can relate the current operator j a and the spin operator σ b as as j a is obtained by replacing k with k + e A and taking derivative of the Hamiltonian with the vector potential A . By using the above relation between σ b and j a , is equal to λσ xy with the coefficient . By taking the variational derivative of A 0 in equation (5) with respect to S x and S y , one can derive the equation of motion and obtain the spin wave gap as , which is equivalent to equation (4) used to fit the data. Thus, the correspondence between E g and σ xy is expected from the fact that the band crossings act as the magnetic monopoles in momentum space. Here we need to assume that K is independent of T to justify the fitting by equation (4). This fact is consistent with the expectation that the Weyl fermion does not resonantly contribute to K , as the energy denominator is ɛ n ( k )– ɛ m ( k ) in equation (10) for K , whereas the expression of α in equation (11) contains the energy denominator ( ɛ n ( k )– ɛ m ( k )) 2 . Data availability The authors declare that the data supporting the findings of this study are available within the article. How to cite this article: Itoh, S. et al . Weyl fermions and spin dynamics of metallic ferromagnet SrRuO 3 . Nat. Commun. 7:11788 doi: 10.1038/ncomms11788 (2016).